Structural analysis of the transitional state of Arp2/3 complex activation by two actin-bound WCAs Actin filament nucleation and branching by Arp2/3 complex is activated by nucleation-promoting factors (NPFs), whose C-terminal WCA region contains binding sites for actin (W) and Arp2/3 complex (CA). It is debated whether one or two NPFs are required for activation. Here we present evidence in support of the two-NPF model and show that actin plays a crucial role in the interactions of two mammalian NPFs, N-WASP and WAVE2, with Arp2/3 complex. Competition between actin–WCA and glia maturation factor (GMF) for binding to Arp2/3 complex suggests that during activation the first actin monomer binds at the barbed end of Arp2. Based on distance constraints obtained by time-resolved fluorescence resonance energy transfer, we define the relative position of the two actin–WCAs on Arp2/3 complex and propose an atomic model of the 11-subunit transitional complex. The proteins that catalyse the formation of new actin filaments in cells, known as actin filament nucleators, play essential roles in the control of cytoskeleton remodelling in processes such as cell motility, vesicle trafficking and endocytosis [1] , [2] , [3] . Filament nucleators overcome the rate-limiting step for polymerization, that is, the formation of actin dimers and trimers [4] , thus determining the time and location for polymerization. Among filament nucleators, Arp2/3 complex is unique in its ability to mediate both nucleation and branching of actin filaments [5] , [6] . Arp2/3 complex consists of seven proteins, including the actin-related proteins 2 and 3 (Arp2 and Arp3), which function as an actin-like dimer during nucleation [7] , [8] . The other subunits, ArpC1–5, mediate regulatory interactions with various cofactors and branching interactions with the mother filament [8] , and form a scaffold for stabilization of the Arp2–Arp3 heterodimer [7] . By itself, Arp2/3 complex is inactive [7] , [9] , [10] . It is activated by multiple inputs, including ATP [11] , the mother filament [12] , and nucleation-promoting factors (NPFs) [9] , [13] . Classical NPFs, such as WASP, N-WASP, WAVE and WHAMM, are generally unrelated, but they all contain a C-terminal WCA ( W H2, C entral, A cidic) region featuring binding sites for actin (W) [14] and Arp2/3 complex (CA) [12] , [15] . The WCA region of NPFs is sufficient to catalyse the nucleation and branching reaction [9] , whereas their other domains are typically implicated in regulation and localization [16] , [17] . WCA brings together ATP–actin and ATP–Arp2/3 complex and induces a conformational change in the complex that promotes side binding to the mother filament [18] and formation of a branch (daughter) filament that grows from the barbed end of the Arps at a 70° angle relative to the mother filament [8] , [10] . Different methods have been used to map the interactions of WCA with Arp2/3 complex, including chemical crosslinking [19] , [20] , [21] , [22] , NMR [19] , [20] , direct interaction of purified proteins [23] , SAXS [24] , transfers of photoactivatable labels [25] and X-ray crystallography [26] . Collectively, these results implicate subunits Arp2, Arp3, ArpC1 and ArpC3 in interactions with WCA. Some of these subunits are >50 Å apart in the inactive complex [7] , which given the short length of the WCA polypeptide is difficult to reconcile with a single WCA-binding site. Two groups have now reported that Arp2/3 complex binds two NPFs [25] , [26] , which leads to more efficient activation and is consistent with the observation that in cells NPFs are frequently clustered on membranes or bound to dimeric partners [27] . However, these reports were recently disputed by a study that found that Arp2/3 complex bound a single NPF [28] . Here we test the two competing models of activation, placing special emphasis on the role of actin in the interaction of WCA with Arp2/3 complex. We conclude that the WCAs of two NPFs, N-WASP and WAVE2, bind with 2:1 stoichiometry to Arp2/3 complex, both in isolation and when bound to actin. Based on competition experiments with glia maturation factor (GMF) and distance measurements by time-resolved fluorescent energy transfer (TR-FRET), we further show that the first actin subunit binds at the barbed end of Arp2 and propose a detailed atomic model of the transitional complex formed by two actin–WCAs and Arp2/3 complex. Preparation of stable actin–WCA complexes In cells, where the concentration of actin monomers is high (>100 μM) [29] , NPFs are likely to be pre-bound to actin, which interacts with relatively high affinity ( K d <1.0 μM) with the W domain [12] , [14] , [30] , [31] . As the actin subunits bound to NPFs are thought to contact the barbed end of Arp2, Arp3 or both, it is likely that NPFs interact differently with Arp2/3 complex depending on whether or not they are pre-bound to actin. However, testing this hypothesis has proven difficult, due to spontaneous polymerization of actin, which interferes with biochemical and structural studies under physiological conditions. While latrunculin (A or B) has been used in some studies to prevent polymerization [25] , [32] , this toxin binds in the nucleotide-binding cleft at the pointed end of the actin monomer and is thus expected to interfere with proper interaction with the Arps, as suggested by a recent study [28] and analogous to its effect on actin–actin interactions [33] . To circumvent these problems, we devised two strategies: crosslinking of actin to WCA and substitution of the N-terminal region of the W domain by gelsolin segment 1 (GS1) ( Fig. 1 ). Both approaches avoid the need for latrunculin, producing highly stable actin–WCA complexes that capture the intermediate polymerization nucleus formed by Arp2/3 complex, WCA and actin. Additionally, both approaches inhibit Arp2/3 complex nucleation, simplifying the analysis. 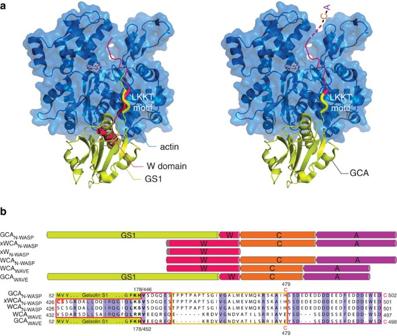Figure 1: Design of WCA constructs. (a) Superimposition of the structures of actin (blue) bound to GS1 (ref. 35)35(yellow, PDB code: 1P8Z) and W14(red, PDB code: 2A3Z), and design of GCA constructs in which the N-terminal portion of W is replaced by GS1. The motif ‘LKKT’, present in both GS1 and the W domain, was used as the fusion site. (b) Schematic representation and sequence of WCA constructs of N-WASP and WAVE2 (W, red; C, orange; A, magenta; GS1, yellow). Residues that were mutated are highlighted in red. N-WASP residues426CS427were mutated to426SC427in constructs xWN-WASPand xWCAN-WASPfor direct, unconstrained crosslinking to actin Cys-374. Single cysteine variants of constructs GCAN-WASP(H479C or C502 added at the C terminus) and GCAWAVE(E479C or C498 added at the C terminus) were made for labelling with fluorophores. Residues in the LKKT motif are highlighted in bold. Figure 1: Design of WCA constructs. ( a ) Superimposition of the structures of actin (blue) bound to GS1 (ref. 35) [35] (yellow, PDB code: 1P8Z) and W [14] (red, PDB code: 2A3Z), and design of GCA constructs in which the N-terminal portion of W is replaced by GS1. The motif ‘LKKT’, present in both GS1 and the W domain, was used as the fusion site. ( b ) Schematic representation and sequence of WCA constructs of N-WASP and WAVE2 (W, red; C, orange; A, magenta; GS1, yellow). Residues that were mutated are highlighted in red. N-WASP residues 426 CS 427 were mutated to 426 SC 427 in constructs xW N-WASP and xWCA N-WASP for direct, unconstrained crosslinking to actin Cys-374. Single cysteine variants of constructs GCA N-WASP (H479C or C502 added at the C terminus) and GCA WAVE (E479C or C498 added at the C terminus) were made for labelling with fluorophores. Residues in the LKKT motif are highlighted in bold. Full size image Crosslinking, which we reported previously [24] , is based on the structures of W domains bound to actin [14] , and takes advantage of the proximity of actin’s reactive Cys-374 to the N-terminal helix of the W domain, in which we introduced a cysteine residue for direct disulphide bond formation ( Fig. 1b ). We determined the crystal structure of a W domain crosslinked to actin in this manner and found it to be nearly identical to those of non-crosslinked W-actin complexes [34] . Here we made two constructs for crosslinking of the WCA and W regions of N-WASP to actin, xWCA N-WASP and xW N-WASP ( Fig. 1 ). Crosslinking, however, has drawbacks; it precludes the use of additional cysteine substitutions for labelling of WCA with fluorophores and impedes the use of reducing agents necessary to stabilize Arp2/3 complex over longer periods of time. Our second approach resolves these shortcomings by taking advantage of the presence of a ‘LKKT’ motif in the linker between gelsolin domains 1 and 2, which is structurally equivalent to that of the W domain [14] , [35] ( Fig. 1a ). Accordingly, we substituted the N-terminal portion of the W domain in the WCAs of N-WASP and WAVE2 with GS1. The resulting constructs are referred to here as GCA N-WASP and GCA WAVE ( Fig. 1 and Supplementary Fig. 1 ). Previously, we found that crosslinking of WCA to actin strongly inhibited nucleation by Arp2/3 complex (20 nM) in the presence of 2 μM actin (6% pyrene-labelled) [24] . Under these conditions, we found here that 200 nM GCA N-WASP has an even stronger inhibitory effect on polymerization ( Supplementary Fig. 2 ). NPFs dissociate from branch junctions immediately after nucleation [36] . GS1, which binds with picomolar affinity to actin [37] and crosslinked WCA do not dissociate, and probably inhibit polymerization by interfering with actin subunit addition at the barbed end of the first two actins. That inhibition is greater for GCA N-WASP than xWCA is consistent with the larger size of GS1, that is, the smaller W domain obstructs, but does not fully block barbed end monomer addition. Two N-WASP WCAs bind to Arp2/3 complex with or without actin There are differences between the two studies that reported interaction of Arp2/3 complex with two WCAs [25] , [26] . Using isothermal titration calorimetry (ITC), one study established that yeast Arp2/3 complex bound two CAs of yeast Wsp1p, but both yeast and mammalian Arp2/3 complex bound only one CA of mammalian N-WASP [26] . This study also concluded that actin–WCA bound with weaker affinity to Arp2/3 complex than CA alone. In contrast, the other study found that the stoichiometry of the mammalian complex was 2:1 (WCA–Arp2/3 complex) in the presence or the absence of actin–latrunculin B [25] . Moreover, these studies were challenged by a work that found that Arp2/3 complex binds a single WCA with or without actin [28] . Here, we tested the two competing models of activation, addressing specifically the role of actin in the interaction of mammalian Arp2/3 complex and NPFs. First, we analysed the binding of WCA N-WASP alone to Arp2/3 complex by ITC, which resulted in an exothermic reaction ( Fig. 2a ) with similar profile to that of yeast Arp2/3 complex with Wsp1p CA [26] . While the reaction was consistent with two WCA-binding sites (inflection point near 1:1 molar ratio), stoichiometry and affinity are interconnected during fitting of ITC data to a binding isotherm. Therefore, different fitting models were tested ( Supplementary Fig. 3 ). In this case, the best fit corresponded to a two-independent-site binding model ( Figs 2a and 3 and Table 1 ). The affinity of site 1 was nearly ninefold higher than that of site 2 ( K d of 20 versus 182 nM), and both affinities were an order of magnitude higher than reported for the yeast complex [26] . 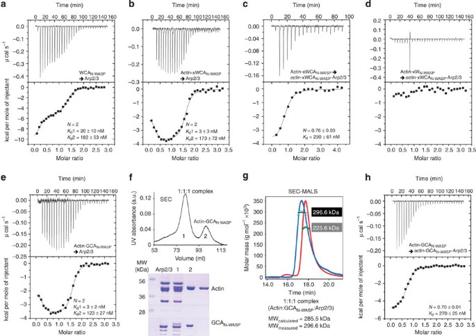Figure 2: Two N-WASP WCAs bind to Arp2/3 complex with or without actin. (a) ITC titration of 157 μM WCAN-WASPinto 10 μM Arp2/3 complex. The best fit of the data corresponded to a two-site binding isotherm (Table 1). The reported errors correspond to the s.d. of the fit. (b) Titration of 189 μM actin–xWCAN-WASPinto 12.5 μM Arp2/3 complex. (c) Titration of 136 μM actin–xWCAN-WASPinto 4 μM 1:1:1 actin–xWCAN-WASP-Arp2/3 complex purified by gel filtration after the experiment shown in partb(Supplementary Fig. 4). (d) Titration of 86 μM actin–xWN-WASPinto 5 μM purified 1:1:1 actin–xWCAN-WASP–Arp2/3 complex. (e) Titration of 147 μM actin–GCAN-WASPinto 9.9 μM Arp2/3 complex. (f) Purification by gel filtration of the saturated complex resulting from the experiment shown ine. Analysis by SDS-PAGE reveals that peak 1 consists of Arp2/3 complex with bound actin–GCAN-WASPand peak 2 consists of actin–GCAN-WASPdissociating from the weak-affinity site 2. (g) SEC-MALS analysis of peak 1 reveals a 1:1:1 actin–GCAN-WASP–Arp2/3 complex with mass 296.6 kDa (blue trace; calculated mass 285.5 kDa). Arp2/3 complex alone is shown as a control (red trace; measured mass 225.6 kDa, calculated mass 223.6 kDa). (h) Titration of 106 μM actin–GCAN-WASPinto 7 μM purified 1:1:1 actin–GCAN-WASP–Arp2/3 complex. Figure 2: Two N-WASP WCAs bind to Arp2/3 complex with or without actin. ( a ) ITC titration of 157 μM WCA N-WASP into 10 μM Arp2/3 complex. The best fit of the data corresponded to a two-site binding isotherm ( Table 1 ). The reported errors correspond to the s.d. of the fit. ( b ) Titration of 189 μM actin–xWCA N-WASP into 12.5 μM Arp2/3 complex. ( c ) Titration of 136 μM actin–xWCA N-WASP into 4 μM 1:1:1 actin–xWCA N-WASP -Arp2/3 complex purified by gel filtration after the experiment shown in part b ( Supplementary Fig. 4 ). ( d ) Titration of 86 μM actin–xW N-WASP into 5 μM purified 1:1:1 actin–xWCA N-WASP –Arp2/3 complex. ( e ) Titration of 147 μM actin–GCA N-WASP into 9.9 μM Arp2/3 complex. ( f ) Purification by gel filtration of the saturated complex resulting from the experiment shown in e . Analysis by SDS-PAGE reveals that peak 1 consists of Arp2/3 complex with bound actin–GCA N-WASP and peak 2 consists of actin–GCA N-WASP dissociating from the weak-affinity site 2. ( g ) SEC-MALS analysis of peak 1 reveals a 1:1:1 actin–GCA N-WASP –Arp2/3 complex with mass 296.6 kDa (blue trace; calculated mass 285.5 kDa). Arp2/3 complex alone is shown as a control (red trace; measured mass 225.6 kDa, calculated mass 223.6 kDa). ( h ) Titration of 106 μM actin–GCA N-WASP into 7 μM purified 1:1:1 actin–GCA N-WASP –Arp2/3 complex. 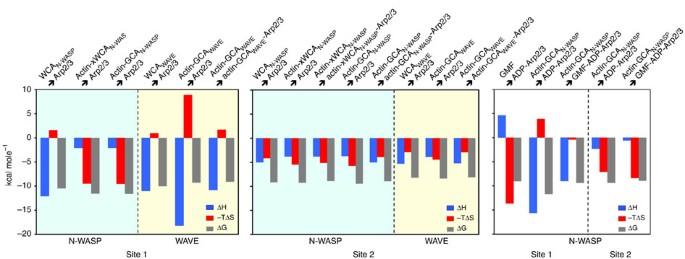Figure 3: Schematic representation of the thermodynamic parameters of Arp2/3 complex interactions with WCA species. Experiments are color-coded: cyan, titrations of WCA variants of N-WASP; yellow, titrations of WCA variants of WAVE2 and white, titrations of GMF and GCAN-WASPinto ADP–Arp2/3 complex. The data is separated into binding sites 1 and 2. Full size image Figure 3: Schematic representation of the thermodynamic parameters of Arp2/3 complex interactions with WCA species. Experiments are color-coded: cyan, titrations of WCA variants of N-WASP; yellow, titrations of WCA variants of WAVE2 and white, titrations of GMF and GCA N-WASP into ADP–Arp2/3 complex. The data is separated into binding sites 1 and 2. Full size image Table 1 Thermodynamic parameters of ITC titrations. Full size table The titration of crosslinked actin–xWCA N-WASP into Arp2/3 complex also fitted best to a two-independent-site model ( Fig. 2b ). In the presence of actin, the affinity of site 2 remained mostly unchanged, while that of site 1 appeared to increase somewhat ( K d of 3 versus 20 nM). However, these high-affinity values fall near the accuracy limits of the ITC instrument ( K d ≤10 nM), and precise comparison is not warranted. It is more informative to compare the thermodynamic parameters of the titrations ( Fig. 3 and Table 1 ). For site 2, we did not observed significant differences in thermodynamic parameters±actin. In contrast, there was a major change in site 1, from an enthalpy-driven reaction in the absence of actin to an entropy-driven reaction in the presence of actin. These results suggest that at least for N-WASP actin has no appreciable contribution to the interaction at site 2, but contributes substantially to the binding energy at site 1. To experimentally validate the 2:1 model used for fitting, saturated actin–xWCA N-WASP -Arp2/3 complex was purified by gel filtration ( Supplementary Fig. 4a ), resulting in separation of two species. Characterization of these species by SDS-PAGE and multi-angle light scattering (MALS) revealed that the first peak consisted of a stable 1:1:1 complex (actin–xWCA N-WASP -Arp2/3 complex) and the second peak corresponded to actin–xWCA N-WASP dissociating from the weaker-affinity site 2 ( Supplementary Fig. 4b ). The 1:1:1 complex corresponds to the one studied by us previously by SAXS [24] , and shows that in that study one actin–xWCA N-WASP was lost during gel filtration. Re-titration of actin–xWCA N-WASP into the purified 1:1:1 complex resulted in binding to a single site, restoring a 2:2:1 actin–xWCA N-WASP -Arp2/3 complex ( Fig. 2c ). The affinity, thermodynamic parameters and profile of the titration show that this binding corresponds to site 2 of the initial titration ( Figs 2b,c and 3 and Table 1 ). Importantly, crosslinked actin–xW N-WASP (lacking CA) did not bind to the purified 1:1:1 complex ( Fig. 2d ), further suggesting that actin does not contribute much to the interaction at site 2. Next, we titrated actin–GCA N-WASP into Arp2/3 complex. The titration and thermodynamic parameters of the reaction were strikingly similar to those observed with actin–xWCA N-WASP ( Figs 2b,e and 3 ). GCA N-WASP and xWCA N-WASP differ only in the way they interact with actin ( Fig. 1 ), and the striking similarity of these two titrations appears to cross-validate both methods of stabilization of WCA complexes with actin. In both cases, the presence of actin led to a dramatic change in the binding isotherm for site 1 (molar ratios≤1). After confirming that dissociation of Arp2/3 complex subunits did not occur during titration ( Supplementary Fig. 5a ), we repeated this experiment using lower protein concentrations to better resolve the transition at site 1. Independent of protein concentration, all the titrations fitted to two-binding-site isotherms, with similar affinities and thermodynamic parameters. As above, the saturated 2:2:1 actin–GCA N-WASP -Arp2/3 complex was purified by gel filtration and analysed by SDS-PAGE and MALS, which again revealed two species: a 1:1:1 complex and actin–GCA N-WASP dissociating from site 2 ( Fig. 2f,g ). The 1:1:1 complex was re-titrated with actin–GCA N-WASP , which bound to a single site, restoring the 2:2:1 complex ( Fig. 2h ). The affinity of the interaction and the thermodynamic parameters and profile of the titration show that this binding corresponds to site 2 of the initial titration ( Figs 2e,h and 3 ). Two WAVE2 WCAs bind to Arp2/3 complex with or without actin To test whether these results could be generalized to other NPFs, we performed similar experiments with WAVE2. The WCA of WAVE2 also bound to two sites on Arp2/3 complex, but the affinities of both sites were lower than for N-WASP ( Fig. 4a ). Similarly, the titration of actin–GCA WAVE fitted best to a two-independent-site model, but with significantly lower affinities than for actin–GCA N-WASP ( Fig. 4b , Table 1 and Supplementary Fig. 3b ). Analysis by MALS of the saturated complex after the ITC titration revealed a reaction boundary ( Fig. 4c ), consistent with complex dissociation. Purification of this complex by gel filtration resulted in two peaks, which by SDS-PAGE corresponded to dissociating actin–GCA WAVE and Arp2/3 complex with a sub-stoichiometric amount of actin–GCA WAVE bound ( Fig. 4d ). Thus, actin–GCA WAVE dissociates during gel filtration not only from site 2 but also partially from site 1, consistent with the lower affinity of this NPF. This was confirmed by re-titrating the purified complex with actin–GCA WAVE , which resulted in two binding sites ( Fig. 4e ). 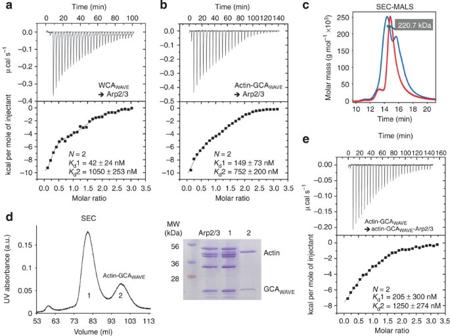Figure 4: Two WAVE2 WCAs bind to Arp2/3 complex with or without actin. (a) Titration of 127 μM WCAWAVEinto 8.9 μM Arp2/3 complex. The best fit of the data corresponded to a two-site binding isotherm (Table 1). The reported errors correspond to the s.d. of the fit. (b) Titration of 167 μM actin–GCAWAVEinto 11 μM Arp/3 complex. (c) Analysis by MALS of the saturated complex after the experiment shown inbreveals a reaction boundary (blue trace) with two peaks on each side of the Arp2/3 complex control (red trace). The masses of these peaks could not be accurately measured. (d) Purification by gel filtration of the saturated complex from the experiment shown inb. Analysis by SDS-PAGE revealed that peak-1 contained Arp2/3 complex and a sub-stoichiometric amount of actin–GCAWAVE, whereas peak-2 contained actin–GCAWAVEdissociating from Arp2/3 complex. Note that in this gel, GCAWAVEoverlaps with subunit ArpC3. (e) The titration of 74.4 μM actin–GCAWAVEinto peak-1 of the gel filtration (at ~4.9 μM) displayed a similar profile as the titration into Arp2/3 complex alone (b) and was best fitted to a two-site binding model. Figure 4: Two WAVE2 WCAs bind to Arp2/3 complex with or without actin. ( a ) Titration of 127 μM WCA WAVE into 8.9 μM Arp2/3 complex. The best fit of the data corresponded to a two-site binding isotherm ( Table 1 ). The reported errors correspond to the s.d. of the fit. ( b ) Titration of 167 μM actin–GCA WAVE into 11 μM Arp/3 complex. ( c ) Analysis by MALS of the saturated complex after the experiment shown in b reveals a reaction boundary (blue trace) with two peaks on each side of the Arp2/3 complex control (red trace). The masses of these peaks could not be accurately measured. ( d ) Purification by gel filtration of the saturated complex from the experiment shown in b . Analysis by SDS-PAGE revealed that peak-1 contained Arp2/3 complex and a sub-stoichiometric amount of actin–GCA WAVE , whereas peak-2 contained actin–GCA WAVE dissociating from Arp2/3 complex. Note that in this gel, GCA WAVE overlaps with subunit ArpC3. ( e ) The titration of 74.4 μM actin–GCA WAVE into peak-1 of the gel filtration (at ~4.9 μM) displayed a similar profile as the titration into Arp2/3 complex alone ( b ) and was best fitted to a two-site binding model. Full size image These results reveal differences and similarities between N-WASP and WAVE. WAVE2’s WCA is 10-aa shorter than that of N-WASP ( Fig. 1b ), with deletions in the C and A regions that might constrain binding to Arp2/3 complex. The shorter length may explain why WAVE2’s WCA has lower affinity for Arp2/3 complex with or without actin ( Figs 2 and 4 ). Also different from N-WASP, the interaction of WAVE2’s WCA with site 1 is enthalpy-driven independent of the presence of actin, whereas that of N-WASP becomes entropy-driven in the presence of actin ( Fig. 3 ). Yet, both NPFs bind with 2:1 stoichiometry to Arp2/3 complex with or without actin. Moreover, when bound to actin, the interactions of both NPFs with site 1 undergo large changes in thermodynamic parameters, whereas the interactions with site 2 are mostly unchanged by actin ( Fig. 3 ). The first actin subunit binds at the barbed end of Arp2 Different studies have distinctly proposed that the first actin subunit binds at the barbed end of Arp2 (refs 24 , 25 , 32 ) or Arp3 (refs 20 , 26 , 38 ), but with the exception of the SAXS analysis of the 1:1:1 actin–xWCA-Arp2/3 complex, which placed the first actin at the barbed end of Arp2 (ref. 24 ), there is no direct evidence in support of either model. To address this question, we used competition between actin–GCA N-WASP and GMF for binding to Arp2/3 complex. The ADF/cofilin-family member GMF interacts with Arp2/3 complex and promotes debranching [39] . We recently found that GMF interacts very weakly with ATP–Arp2/3 complex but forms a relatively tight 1:1 complex with ADP–Arp2/3 complex [40] . A recent structure showed that GMF binds at the barbed end of Arp2 (ref. 41 ). We reasoned that if the first actin subunit binds at the barbed end of Arp2, it should compete with GMF binding. To test this idea, we first established that actin–GCA N-WASP could bind ADP–Arp2/3 complex ( Fig. 5a ). At saturation, the stoichiometry of the interaction was 2:2:1 actin–GCA N-WASP -Arp2/3 complex, and the affinities of both sites were similar to those observed in the ATP state. In contrast, we observed a dramatic change in the character of the interaction at site 1, from entropy-driven binding in the ATP state to enthalpy-driven binding in the ADP state ( Fig. 3 and Table 1 ). As the only difference between these experiments is the nucleotide state of Arp2/3 complex (actin retains the bound ATP after dialysis, Methods), this finding is consistent with a nucleotide-dependent conformational change in Arp2/3 complex [11] . Purification by gel filtration of the 2:2:1 complex formed in the ADP state produced two species, identified by SDS-PAGE and MALS as a 1:1:1 actin–GCA N-WASP -Arp2/3 complex (measured mass 282.5 kDa) and actin–GCA N-WASP dissociating from the lower-affinity site 2 ( Fig. 5b ). As before [40] , GMF-bound ADP-Arp2/3 complex with a K d ~0.2 μM ( Supplementary Fig. 6 ). However, GMF did not bind to the purified 1:1:1 complex ( Fig. 5c ), suggesting direct competition with actin–GCA N-WASP for binding to Arp2. 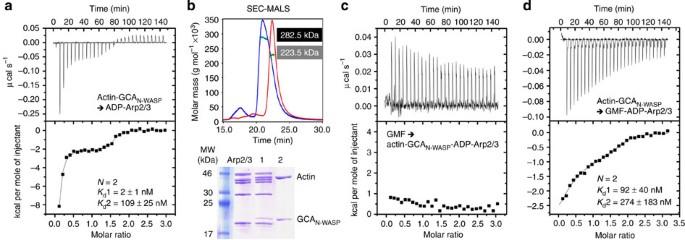Figure 5: Competition between GMF and GCAN-WASPfor binding to ADP–Arp2/3 complex. (a) Titration of 112 μM actin–GCAN-WASPinto 8.0 μM ADP–Arp/3 complex. The best fit of the data was to a two-site binding isotherm (Table 1). The reported errors correspond to the s.d. of the fit. (b) Analysis by MALS and SDS-PAGE of the two species resulting from gel filtration (not shown) of the saturated complex after the experiment shown ina. Peak-1 consisted of a 1:1:1 actin–GCAN-WASP–Arp2/3 complex in the ADP state (blue trace; measured mass 282.5, calculated mass 285.5 kDa) and peak-2 contains actin–GCAN-WASPdissociating from site 2. Arp2/3 complex alone is shown as a control (red trace). (c) Titration of 90 μM GMF into 6.3 μM purified 1:1:1 actin–GCAN-WASP–Arp2/3 complex (b, peak-1). (d) Titration of 107 μM actin–GCAN-WASPinto 7.7 μM saturated GMF–Arp/3 complex (from the experiment shown inSupplementary Fig. 6). Figure 5: Competition between GMF and GCA N-WASP for binding to ADP–Arp2/3 complex. ( a ) Titration of 112 μM actin–GCA N-WASP into 8.0 μM ADP–Arp/3 complex. The best fit of the data was to a two-site binding isotherm ( Table 1 ). The reported errors correspond to the s.d. of the fit. ( b ) Analysis by MALS and SDS-PAGE of the two species resulting from gel filtration (not shown) of the saturated complex after the experiment shown in a . Peak-1 consisted of a 1:1:1 actin–GCA N-WASP –Arp2/3 complex in the ADP state (blue trace; measured mass 282.5, calculated mass 285.5 kDa) and peak-2 contains actin–GCA N-WASP dissociating from site 2. Arp2/3 complex alone is shown as a control (red trace). ( c ) Titration of 90 μM GMF into 6.3 μM purified 1:1:1 actin–GCA N-WASP –Arp2/3 complex ( b , peak-1). ( d ) Titration of 107 μM actin–GCA N-WASP into 7.7 μM saturated GMF–Arp/3 complex (from the experiment shown in Supplementary Fig. 6 ). Full size image To check that the lack of binding of GMF was not due to long-range allosteric effects, we inverted the order of the titration; actin–GCA N-WASP was titrated into the 1:1 complex of GMF with ADP–Arp2/3 complex ( Fig. 5d ). This resulted in a ~46-fold drop in the affinity of actin–GCA N-WASP for site 1 and large changes in thermodynamic parameters ( Fig. 3 and Table 1 ), whereas the affinity of site 2 decreased only 2.5-fold and the thermodynamic parameters were mostly unchanged. The affinity of actin–GCA N-WASP for site 1 in the ADP state is nearly two orders of magnitude higher than that of GMF ( K d 2 versus 200 nM, Fig. 5a and Supplementary Fig. 6 ), such that it was expected that actin–GCA N-WASP would displace GMF from the complex. Yet, the large changes in thermodynamic parameters and affinity for site 1 strongly suggest that GMF competes with actin–GCA N-WASP for binding to this site, and thus the first actin subunit most likely binds at the barbed end of Arp2. Steady-state FRET confirms two actin–WCA-binding sites To independently test the two-site binding model, we used steady-state FRET. Cysteine residues were introduced by mutagenesis at the end of the C region or added C-terminally to the A region in constructs GCA N-WASP and GCA WAVE ( Fig. 1b ). We refer to these two labelling sites as positions 1 for the donor (or 1′ for the acceptor) and 2 (or 2′), respectively. These mutants were labelled with either the donor probe IAEDANS or the acceptor probe DABMI, a fluorescence pair sensitive to energy transfer in the distance range ~30–65 Å. For each experiment, actin–GCA N-WASP –Arp2/3 complex (or actin–GCA WAVE –Arp2/3 complex) labelled with IAEDANS at position 1 or 2 was pre-purified as described above ( Figs 2f and 4d ) and titrated with actin–GCA N-WASP (or actin–GCA WAVE ) labelled at position 1′ or 2′ with DABMI. Binding to Arp2/3 complex did not change the donor fluorescence, and quenching only occurred in the presence of DABMI-labelled GCA for all the combinations of probe positions in both N-WASP ( Fig. 6a ) and WAVE2 ( Supplementary Fig. 7 ). Additionally, a significant shift toward longer wavelengths (red shift) was observed in all the titrations. A red shift of IAEDANS signal corresponds to a more solvent-exposed environment of the probe [42] , consistent with a conformational change taking place in Arp2/3 complex upon binding of actin–WCA to site 2. The occurrence of a red shift precludes accurate quantitative analysis, yet tentative affinity values for site 2 were obtained by fitting the titrations with the smallest red shift, corresponding to positions 2 and 1′ ( Fig. 6b , Supplementary Fig. 7c ). The resulting affinities appeared underestimated compared with the more reliable values obtained by ITC ( K d values 7 μM versus ~200 nM for actin–GCA N-WASP and 14 μM versus ~1 μM for actin–GCA WAVE ). While these affinities are unreliable due to the red shift and effects of the probes on binding, this analysis confirms the presence of a second binding site for actin–WCA. 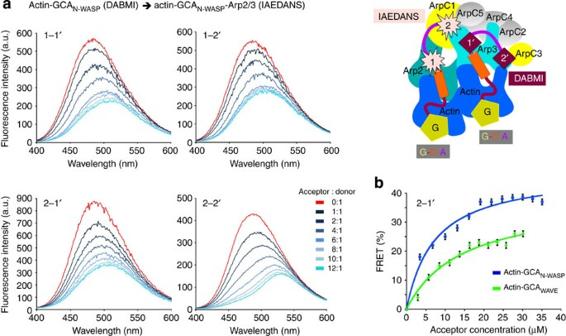Figure 6: Steady-state FRET analysis of actin–GCA binding to Arp2/3 complex. (a) Fluorescence quenching during titration of acceptor-labelled actin–GCAN-WASPinto donor-labelled 1:1:1 actin–GCAN-WASP-Arp2/3 complex. Probe sites and titration ratios are indicated. A cartoon representation illustrates the relative positions of the donor (IAEDANS) and acceptor (DABMI) probes in these experiments. (b) FRET as a function of acceptor concentration for the 2–1′ titrations (with smallest red shift) of actin–GCAN-WASP(blue) and actin–GCAWAVE(green, experiment shown inSupplementary Fig. 7). Data points represent mean±s.e.m. from three independent measurements. Data fitting resulted inKdvalues of 7 and 14 μM for actin–GCAN-WASPand actin–GCAWAVE, respectively. Figure 6: Steady-state FRET analysis of actin–GCA binding to Arp2/3 complex. ( a ) Fluorescence quenching during titration of acceptor-labelled actin–GCA N-WASP into donor-labelled 1:1:1 actin–GCA N-WASP -Arp2/3 complex. Probe sites and titration ratios are indicated. A cartoon representation illustrates the relative positions of the donor (IAEDANS) and acceptor (DABMI) probes in these experiments. ( b ) FRET as a function of acceptor concentration for the 2–1′ titrations (with smallest red shift) of actin–GCA N-WASP (blue) and actin–GCA WAVE (green, experiment shown in Supplementary Fig. 7 ). Data points represent mean±s.e.m. from three independent measurements. Data fitting resulted in K d values of 7 and 14 μM for actin–GCA N-WASP and actin–GCA WAVE , respectively. Full size image Relative position of two WCAs on Arp2/3 complex by TR-FRET The observation of energy transfer for all the probe positions opened the way for TR-FRET experiments to determine distances between probes in the complex. In these experiments, we used actin–GCA N-WASP –Arp2/3 complex that can be purified with 1:1:1 stoichiometry (that is, site 1 is fully occupied). A pre-purified 1:1:1 complex containing the donor IAEDANS at position 1 or 2 was mixed with actin–GCA N-WASP containing the acceptor DABMI at one of the two labelling positions. All four possible inter-probe distances (1–1′, 1–2′, 2–1′ and 2–2′) were determined by fitting the fluorescence decays using a double-exponential function ( Supplementary Fig. 8 and Methods). All the distances were tightly clustered in the range 53.8–60.4 Å ( Table 2 ). Table 2 Distances from time-resolved FRET and model. Full size table Another distance constraint was obtained using a double mutant of GCA N-WASP labelled at Cys-479 and Cys-502 with the donor and acceptor probes ( Fig. 1b ). This distance could be only measure for site 1, using the purified 1:1:1 complex, since the saturation state of site 2 cannot be precisely determined, and any unbound actin–GCA N-WASP would contribute to the fluorescence. Double labelling of GCA N-WASP was carried out by under-labelling with IAEDANS, followed by labelling with DABMI (Methods), which produces a mixture of donor–donor, acceptor–acceptor and donor–acceptor species. This mixture was analysed by reverse-phase HPLC, which together with a recording of DABMI absorbance at 502 nm, detection of IAEDANS fluorescence in the peak fractions and deconvolution of the 280 nm absorbance profile, resulted in a 32% estimate of the relevant donor-acceptor fraction ( Supplementary Fig. 9a,b ). To determine the distance between probes, we fitted the donor–acceptor decay using a linear combination of two double-exponential functions ( Supplementary Fig. 9c ), fixing the molar fraction of the donor-acceptor decay to 32%. This analysis resulted in a distance estimate of 47.5 Å between the two probes at site 1. The ensemble of FRET distances provides key constraints for modelling of two WCAs on the surface of Arp2/3 complex. Despite ~20 years of intensive investigation since the discovery of Arp2/3 complex [43] , only recently was it found that optimal activation requires two NPFs [25] , [26] , [27] . This fact was difficult to uncover, first because in isolation most NPFs appear to be monomeric, but also because formation of the short-lived transitional complex is a multi-step and multi-factorial process that requires NPFs, ATP, actin monomers and culminates with binding to the mother filament [44] . The two-NPF model accounts for the fact that multiple binding partners of NPFs are dimeric, and that clustering at membranes would allow for two NPFs to synergistically activate Arp2/3 complex [27] . Strikingly, reinterpretation of most of the published data is also consistent with the two-NPF model [25] . This includes studies showing that subunits Arp2, Arp3, ArpC1 and ArpC3, which are distantly separated in the structure [7] , can all be crosslinked to NPFs [19] , [20] , [21] , [22] . Photoactivatable biotin coupled to cysteine residues along the CA polypeptide also transfers onto these four subunits [25] . Spin labels at the end of the C and A regions causes NMR line broadening of ArpC3 resonances, suggesting that these labels fall within ~25 Å of ArpC3 (ref. 20 ). Recombinant ArpC1 binds WCA, and this interaction depends on the presence of the conserved tryptophan at the end of the A region [23] . SAXS analysis of a 1:1:1 actin–xWCA–Arp2/3 complex places the first actin subunit at the barbed end of Arp2 (ref. 24 ). X-ray crystallography shows three residues of the A region of N-WASP, 502 EWE 504 , bound to Arp3 (ref. 26 ). Collectively, these studies implicate subunits Arp2, Arp3, ArpC1 and ArpC3 in interactions with NPFs, which can only be explained by the two-NPF model. This model also explains how cortactin NTA and N-WASP WCA can co-bind Arp2/3 complex [21] . Despite these considerations, the two-NPF model was challenged by a study that found that Arp2/3 complex interacts with a single NPF with or without actin [28] . The ongoing debate, and the fact that our own SAXS analysis of the 1:1:1 complex [24] was used as supporting evidence in the latter study, motivated us to analyse the two competing models of Arp2/3 complex activation. The results presented here provide strong evidence in support of the two-NPF model, and extend beyond this debate to also provide a likely pathway of the activation reaction and a testable atomic model of the transitional complex. Thus, we established that the WCAs of two mammalian NPFs, N-WASP and WAVE2, both bind mammalian Arp2/3 complex with 2:1 stoichiometry. In the presence of actin, the stoichiometry of the interaction is also 2:2:1. Actin has little effect on the affinity of site 2, but changes the affinity and thermodynamic parameters of site 1 in an NPF-dependent manner. The 2:2:1 stoichiometry is further demonstrated by purification of a half-saturated 1:1:1 complex that can bind a second actin–NPF. Actin–GCA N-WASP binds Arp2/3 complex in the ADP state, interacting with two sites and with similar affinities as in the ATP state, but with markedly different thermodynamic parameters at site 1, consistent with a nucleotide-dependent conformational change [11] . The similar affinity of actin–WCA for ADP– and ATP–Arp2/3 complex is consistent with the finding that ATP hydrolysis is not required for NPF release [36] . GMF, which binds at the barbed end of Arp2 (ref. 41 ), competes with the binding of actin–GCA N-WASP to site 1, suggesting that the first actin subunit is delivered at the barbed end of Arp2. Fluorescence energy transfer between donor-acceptor probes on two actin–GCAs independently confirms the 2:2:1 stoichiometry of the interaction, and reveals a major red shift upon saturation of site 2, consistent with a conformational change. Finally, we obtained a set of five inter-probe distances that combined with published data allow us to build an atomic model of the transitional complex. To build this model ( Fig. 7 and Supplementary Movie 1), we started with the structure of inactive Arp2/3 complex containing three amino acids of the A region bound to Arp3 (ref. 26 ). Arp2, which is partially disordered in this and other structures [7] , [45] , was taken from the structure of the complex with GMF in which it was visualized [41] . In the inactive conformation, Arp2 obstructs binding to the barbed end of Arp3, which is a strong argument in favour of a movement of Arp2 as a first step during activation [24] , [25] . For this, we superimposed the highest-resolution model of the actin filament [46] onto subunit Arp3, which defines the expected position of Arp2 upon activation, as well as those of the first two actin subunits at the barbed ends of Arps. The only conformational change required is a rotation of Arp2, which does not generate steric clashes [24] . The structure of W bound to actin [14] was then superimposed onto the actin subunits at the barbed ends of Arp2 and Arp3. In the structure of Arp2/3 complex, a helix of ArpC1 (residues 297–305) of a symmetry-related complex makes a crystal packing contact with Arp3, which is thought to mimic binding of the C region to Arp3 (ref. 26) [26] . Consistently, this helix, which is conspicuously detached from the rest of ArpC1 ( Fig. 7 ), is proposed to mediate similar contacts with an actin subunit of the mother filament [7] , [8] . Moreover, like the helix in the C-region [47] , the ArpC1 helix has an amphiphilic character, and its hydrophobic side faces Arp3, analogous to the interactions of several actin–binding proteins with actin [48] , [49] . We thus built a model of CA bound to Arp3 (site 2), by superimposing the helix of the C region onto the ArpC1 helix [26] , and finding a likely path for the acidic linker between this helix and 498 EWE 500 (mouse N-WASP numbering) along a positive surface on Arp3. The helix of the C-region was assumed to bind to Arp2 (site 1) in a way analogous to its interaction with Arp3, with the remaining, non-helical portion of the C-region extending toward the pointed end of Arp2. To this point, our model is in agreement with that proposed by Padrick et al. [25] , and overlaps with two other models regarding the interactions of CA with Arp2 (ref. 24 ) and Arp3 (ref. 26 ). We also observe a strong correlation between experimentally measured FRET distances for probe pairs at positions 1–1′ and 1–2′ and the corresponding distances between Cα atoms in the model ( Fig. 7 and Table 2 ). 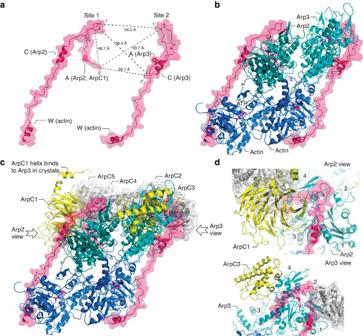Figure 7: Model of the transitional complex formed by Arp2/3 complex, two actin subunits and two WCAs. The PDB codes of the structures used to build this model are: Arp2/3 complex (3RSE), Arp2 (4JD2) and W-actin (2A3Z). (a) Two WCAs in their proposed Arp2/3 complex-bound conformation, showing the distances between Cα atoms of residues labelled in FRET experiments. (b) Proposed pseudo-symmetric interaction of two WCAs with Arp2–actin and Arp3–actin arranged in a filament-like conformation. (c) Illustration of the 11-subunit transitional complex. Subunits ArpC1 and ArpC3, which biochemical data place near the binding site of WCAs, are coloured yellow. Subunits ArpC2, ArpC4 and ArpC5, thought not to interact with NPFs, are coloured grey. (d) Close-up views of sites 1 (Arp2-ArpC1) and site 2 (Arp3-ArpC3). Subdomains 1–4 of Arp2 and Arp3 are indicated. See also Supplementary Movie 1. Figure 7: Model of the transitional complex formed by Arp2/3 complex, two actin subunits and two WCAs. The PDB codes of the structures used to build this model are: Arp2/3 complex (3RSE), Arp2 (4JD2) and W-actin (2A3Z). ( a ) Two WCAs in their proposed Arp2/3 complex-bound conformation, showing the distances between Cα atoms of residues labelled in FRET experiments. ( b ) Proposed pseudo-symmetric interaction of two WCAs with Arp2–actin and Arp3–actin arranged in a filament-like conformation. ( c ) Illustration of the 11-subunit transitional complex. Subunits ArpC1 and ArpC3, which biochemical data place near the binding site of WCAs, are coloured yellow. Subunits ArpC2, ArpC4 and ArpC5, thought not to interact with NPFs, are coloured grey. ( d ) Close-up views of sites 1 (Arp2-ArpC1) and site 2 (Arp3-ArpC3). Subdomains 1–4 of Arp2 and Arp3 are indicated. See also Supplementary Movie 1. Full size image No detailed model has yet been proposed for the A region at site 1. However, it has been abundantly documented that this region contacts both Arp2 and ArpC1 (refs 19 , 20 , 21 , 22 , 23 , 25 ). Therefore, our model must explain this data, while also accounting for the FRET distances. Many models were tested. Models that placed the A region on the exposed surface of ArpC1 produced distances >90 Å for the probe at position 2, whereas models in which the A region was directed toward Arp3 resulted in distances <30 Å for this probe. These models were rejected, since these distances would not be measurable using our FRET pair. Other models in which the A region was directed toward subunits ArpC2, ArpC4 and ArpC5 were not only inconsistent with the biochemical data, but invariably also failed to satisfy the ensemble of the FRET distances. Surprisingly, the only model that satisfied all the criteria was based on the concept of pseudo-symmetry in the way CA interacts with Arp2 and Arp3 ( Fig. 7 , Table 2 and Supplementary Movie 1). In this model, the A region threads through a channel at the interface between Arp2 and ArpC1. Importantly, when CA first encounters Arp2 and ArpC1 in the inactive complex, these two subunits are separated and the binding surface is fully exposed on both sides. In other words, this model predicts that the A region adds affinity between Arp2 and ArpC1 by creating a new binding interface between these two subunits. As a final step, the stereochemistry of the resulting 11-subunit transitional complex (Arp2/3 complex, 2 actin subunits and 2 WCAs) was regularized using the program Phenix [50] . While the model satisfies the FRET constraints and accounts for published data, it is important to understand its limitations. First, it is based on the assumption that during activation the overall structure of the complex remains mostly unchanged, except for the position of Arp2 and smaller changes at the interface between actin–WCA and Arp2, ArpC1 and Arp3. It is likely that other changes occur, particularly at the interface with the mother filament. The model is also based on the assumption that Arp2, Arp3 and the actin subunits bound at their barbed ends adopt a filament-like conformation. However, deviations from this structure are likely, particularly that the filament model is only defined to limited (non-atomic) resolution [46] . Finally, while we have aimed to satisfy FRET distances, these distances contain measurement and fitting errors and the position of the fluorophores is not precisely determined. Nevertheless, the proposed atomic model accounts for the overwhelming majority of the published data [19] , [20] , [21] , [22] , [23] , [24] , [25] , [26] , [27] and will be available for independent testing. Because, at both sites the CA polypeptide meanders near the pointed ends of Arp2 and Arp3, this model also accounts for EM data showing extra density at the pointed ends of the Arps when WCA is bound to Arp2/3 complex [51] . This is also the surface that contacts the mother filament in the branch [8] , suggesting that steric hindrance of CA with the mother filament and W with subunits adding to the branch may together trigger NPF dissociation. As proposed above, steric hindrance with subunits adding to the branch may also explain how GCA traps the transitional complex and blocks Arp2/3 complex nucleation, which can now be illustrated by superimposing GS1-actin onto the first two actin subunits of the transitional complex ( Supplementary Fig. 10 ). This superimposition also illustrates that GS1 does not obstruct interactions of the first two actins with Arp2/3 complex or with each other. In summary, based on the ensemble of the results presented here we propose the following sequence of events. Two actin–NPFs bind to Arp2 and Arp3 in a pseudo-symmetric manner. Competition with GMF demonstrates that actin–NPF binds first to Arp2 and ArpC1 (site 1), adding an actin subunit at the barbed of Arp2. This produces a partial conformational change that frees the barbed end of Arp3, allowing for the binding of a second actin–NPF to Arp3. Steady-state FRET shows that this second binding event also leads to a conformational change, which is anticipated to complete the transition of Arp2 and Arp3 into a filament-like conformation and promote binding of Arp2/3 complex to the mother filament. Proteins Arp2/3 complex was purified from bovine brain [24] . Briefly, frozen brains were homogenized in Arp buffer (20 mM HEPES (pH 7.5), 100 mM KCl, 1 mM MgCl 2 , 1 mM EGTA and 1 mM DTT) supplemented with protease inhibitors and clarified by centrifugation at 12,000 g for 30 min. The supernatant was loaded onto a Macro-Prep High Q column (Bio-Rad) pre-equilibrated with Arp buffer. The flow-through, containing Arp2/3 complex, was applied onto a WCA affinity column equilibrated with Arp buffer. Arp2/3 complex was eluted in 20 mM Tris (pH 8.0), 25 mM KCl, 400 mM MgCl 2, 1 mM EGTA and 1 mM DTT, concentrated and further purified through an SD200HL 26/600 column in Arp buffer. Actin was purified from rabbit skeletal muscle [52] . Briefly, an F-actin pellet was homogenized in G-buffer (2 mM Tris (pH 8.0), 0.2 mM CaCl 2 , 0.2 mM ATP and 0.01% NaN 3 ) with the addition of 10 mM DTT to reduce actin fully. After 1 h, actin was dialyzed exhaustively against G-buffer to remove DTT and then centrifuged for 45 min at 277,000 g to pellet any F-actin that did not depolymerize and any denatured actin. The cDNA encoding for mouse N-WASP (UniProt Q91YD9) was obtained from ATCC (clone 3169027). Construct WCA N-WASP was amplified by PCR and cloned between the NdeI and EcoRI sites of vector pTYB12 (New England BioLabs), comprising a chitin-binding domain for affinity purification and an intein domain for self-cleavage after purification (primers listed in Supplementary Table 1 ). Mutations S426C and C427S in construct xWCA N-WASP were introduced with the forward primer during cloning. Construct xW N-WASP , carrying mutations S426C and C427S, was synthesized. The cDNA for expression of mouse WCA WAVE (UniProt Q8BH43) was synthesized (Genewiz) and cloned as above. The cDNA encoding for human gelsolin (UniProt P06396) was purchased from ATCC (clone MGC-39262), and segment 1 (GS1) was cloned as above. The hybrid constructs GCA N-WASP and GCA WAVE were obtained by introducing silent mutations in the GS1 and CA genes that introduced NpsI restriction sites for hybridization in the reverse and forward primers, respectively. The ligation products were then cloned as above. Point mutations H479C in GCA N-WASP and E479C in GCA WAVE were introduced using the QuickChange mutagenesis kit (Qiagen). C-terminal cysteine residues were introduced into constructs GCA N-WASP (Cys-502) and GCA WAVE (Cys-498) using the reverse primers during cloning. The cDNA encoding for human GMFγ (UniProt O60234) was synthesized (Genewiz) and cloned between the NdeI and SapI sites of the pTYB1 vector (New England Biolabs) [40] . All the proteins were expressed in BL21(DE3) cells (Invitrogen), grown in Terrific Broth medium at 37 °C until the OD 600 reached a value of 1.5–2. Expression was induced with 0.5 mM isopropylthio-β-D-galactoside and carried out for 16 h at 20 °C. Cells were harvested by centrifugation, re-suspended in 20 mM HEPES (pH 7.5), 500 mM NaCl, 1 mM EDTA and 100 μM PMSF and lysed using a microfluidizer (Microfluidics). All the proteins were first purified on a chitin affinity column, followed by additional purification as follows: WCA constructs were purified by HPLC using a reverse-phase C18 column and a 0–90% gradient of CH 3 CN in 0.1% TFA, GCA constructs were purified through an ion exchange MonoQ column (Pharmacia) in 20 mM HEPES (pH 7.5) and a 50–1000, mM NaCl gradient and GMFγ was purified by gel filtration on a SD200HL 26/600 column in Arp buffer. Protein concentration was determined spectrophotometrically, using calculated extinction coefficients: 234,080 M −1 cm −1 (Arp2/3 complex), 26,930 M −1 cm −1 (GCA N-WASP ), 28,420 M −1 cm −1 (GCA WAVE ), 5,500 M −1 cm −1 (WCA N-WASP ), 6,990 M −1 cm −1 (WCA WAVE ) and 12,950 M −1 cm −1 (GMFγ). Labelling with fluorophores Cysteine mutants of GCA constructs were reduced with 20 mM DTT for 30 min at room temperature. DTT was removed on a PD10 column (GE Healthcare) in 20 mM HEPES (pH 7.5), 100 mM NaCl and 10 mM EDTA. Single labelling was performed overnight, at 4 °C in the dark, using a 20-fold molar excess of 1,5-IAEDANS or DABMI (Molecular Probes) in the presence of 0.1 mM TCEP. The reaction was stopped by addition of 10 mM DTT. Unreacted probe was removed on a Sephadex G-50 column (GE Healthcare). Labelling was confirmed by mass spectrometry on a Voyager DE-PRO (Applied Biosystems). Double-labelled GCA N-WASP was prepared by labelling first with a 10-fold molar excess of 1,5-IAEDANS (less-reactive probe) for 3 h at room temperature. Unreacted probe was removed as above. Partially labelled GCA N-WASP was then incubated with a 20-fold molar excess of DABMI overnight at 4 °C in the dark. After removal of unreacted probe, double-labelled GCA N-WASP was analysed by HPLC on a reverse-phase C18 analytical column (Waters) using a 0–90% CH 3 CN gradient and 0.1% TFA. The multi-component spectrum was de-convoluted using the program Origin ( Supplementary Fig. 9 ). Complexes of WCA variants with actin and Arp2/3 complex Crosslinked complexes were prepared by mixing actin with xWCA N-WASP or xW N-WASP at a 1.2:1 ratio, using 5,5′-dithiobis(2-nitrobenzoic acid) to facilitate the crosslinking reaction [24] , [34] . Excess actin was then removed on a SD200HL 26/600 column in 20 mM HEPES (pH 7.5), 100 mM KCl, 2 mM MgCl 2, 1 mM EGTA and 0.2 mM ATP. To prepare actin–GCA complexes, actin was mixed with a 1.5 molar excess of GCA N-WASP or GCA WAVE , followed by purification through an SD200HL 26/600 in Arp buffer (with 0.2 mM ATP). The same protocol was used to purify 1:1:1 complexes of labelled actin–GCA bound to Arp2/3 complex. Isothermal titration calorimetry ITC measurements were carried out on a VP-ITC apparatus (MicroCal). Samples were dialyzed for 2 days against Arp buffer (with either 0.2 mM ATP or ADP). Titrations were done at 25 °C (ATP state) or 20 °C (ADP state), the latter temperature being optimal for analysis of endothermic binding of GMFγ [40] . Titrations consisted of 10 μl injections, lasting for 10 s and spaced 300 s apart. The concentration (specified in figures) of the titrant was ~14-fold higher than that of the binding partner in the 1.44 ml cell. The heat of binding was corrected for the small exothermic heat of injection, determined by injecting ligand into buffer. Data were analysed using the program Origin (OriginLab Corporation). In competition experiments with GMF, actin–GCA N-WASP and Arp2/3 complex were dialyzed side-by-side for 2 days against Arp buffer supplemented with 0.2 mM ADP, resulting in ADP incorporation into Arp2/3 complex (purified Arp2/3 complex has no nucleotide bound [45] ), but not actin. Indeed, actin bound to GS1 does not exchange nor hydrolyze the bound ATP, unless hexokinase and glucose are added to the dialysis buffer, which we verified through determination of the crystal structure. Size-exclusion chromatography–multi-angle light scattering For SEC–MALS, samples (100 μl at 1–2 mg ml −1 ) were fractionated on a TSK-gel Super SW2000 column (Tosoh Bioscience) coupled to an Agilent 1100 HPLC system (Agilent Technologies). The molecular species separated by the column were analysed through a DAWN HELEOS MALS detector and an Optilab rEX refractive index detector and their masses calculated with program Astra (Wyatt Technology). Steady-state FRET Steady-state fluorescence emission spectra ( λ em =400–600 nm) were recorded on a Cary Eclipse fluorometer (Varian) with excitation at λ ex =337 nm. DABMI-labelled actin–GCA complexes at 300 μM were titrated into 300 μl of 3 μM pre-purified, IAEDANS-labelled actin–GCA-Arp2/3 complex and incubated for 10 min prior to measurements. Experiments were performed in Arp buffer (with 0.2 mM ATP) at 15 °C. Final spectra were corrected for dilution. Data were fitted using the equation F(x)=F max x/(K d +x) with the program KaleidaGraph (Synergy Software). Time-resolved FRET (TR-FRET) Fluorescence decays were recorded using a TimeMaster T-4 stroboscope lifetime fluorometer (Photon Technology International) with excitation at λ ex =337 nm and emission at λ em =497 nm. Donor fluorescence decays, F D ( t ), were fitted with the function F D,fit ( t ), consisting of the convolution of a multi-exponential decay, F D ( t ), with the instrument response function determined from light scattering by water, where τ Di is the donor-only fluorescence lifetime. In all cases, F D ( t ) was best fitted to two exponentials, n =2 in Equation 1 ( Supplementary Fig. 8 ). The observed fluorescence decays of labelled actin–GCA bound to Arp2/3 complex F D+A ( t ) can be assumed to be a linear combination of fluorescence decays from uncoupled donors, F D ( t ), and donors coupled to acceptors, F DA ( t ). The acceptor is assumed to increase the fluorescence decay rate only through energy transfer. In this case, F D+A ( t ) is fitted by F D+A,fit ( t ): where τ DAi is the fluorescence lifetime of the donor in the presence of the acceptor. All the donors were assumed to be coupled to acceptors in intermolecular FRET samples, and therefore the mole fraction of donor only, X D , was set to 0, and the best fit was obtained with n =2. In the case of intramolecular FRET samples, X D was varied in the fit defined by Equation 2, and n was set to 4 ( Supplementary Fig. 9 ). Distances were calculated from the average donor τ D and donor-acceptor τ DA lifetimes, defined as τ =Σα i τ i 2 /Σα i τ I , according to Equation 3, where R DA is the calculated separation between the donor and acceptor dipoles and R 0 is the Förster distance defined by, where Q D is the quantum yield, κ 2 is the orientation factor (assumed to be 2/3), n is the refractive index of protein in aqueous solution (1.4) and J is the overlap integral between the donor emission and acceptor absorption spectra. The quantum yield was determined at λ ex =350 nm by comparison with a solution of quinine sulphate (1–5 μM in 0.1 M H 2 SO 4 ), with absolute quantum yield of 0.7 (ref. 53 ). Fluorescence decays for intermolecular FRET were analysed using the program FeliX32 (PTI), and decays for intramolecular FRET were analysed with the program FargoFit [54] . How to cite this article: Boczkowska, M. et al. Structural analysis of the transitional state of Arp2/3 complex activation by two actin-bound WCAs. Nat. Commun. 5:3308 doi: 10.1038/ncomms4308 (2014).